Stable silicon-ionic liquid interface for next-generation lithium-ion batteries We are currently in the midst of a race to discover and develop new battery materials capable of providing high energy-density at low cost. By combining a high-performance Si electrode architecture with a room temperature ionic liquid electrolyte, here we demonstrate a highly energy-dense lithium-ion cell with an impressively long cycling life, maintaining over 75% capacity after 500 cycles. Such high performance is enabled by a stable half-cell coulombic efficiency of 99.97%, averaged over the first 200 cycles. Equally as significant, our detailed characterization elucidates the previously convoluted mechanisms of the solid-electrolyte interphase on Si electrodes. We provide a theoretical simulation to model the interface and microstructural-compositional analyses that confirm our theoretical predictions and allow us to visualize the precise location and constitution of various interfacial components. This work provides new science related to the interfacial stability of Si-based materials while granting positive exposure to ionic liquid electrochemistry. While rechargeable lithium-ion batteries (LIBs) have dominated the portable electronics market for nearly a decade, they have failed to gain widespread commercial success in high-power and high-capacity applications. Industry and academia alike have been unable to develop a battery capable of meeting the growing societal and environmental demand for safe, high energy-density, long-lasting energy storage systems [1] , [2] , [3] , [4] , [5] . Such systems could serve to expedite a smooth transition to an electrified transportation market and enable intermittent renewable energy resources, both of which have been gaining attention in our increasingly carbon-constrained world. The search is on for the next generation of electrode materials that will meet such guidelines in a cost effective and efficient manner [6] , [7] , [8] . Recently, silicon has been identified as one of the most attractive high-energy anode materials for LIBs. Silicon’s low working voltage and high-theoretical specific capacity of 3,579 mAh g −1 , nearly ten times higher than that of state-of-the-art graphite anodes, have encouraged widespread research efforts aimed at developing a viable Si-based electrode [9] , [10] , [11] , [12] . The substantial gains in specific and volumetric capacity simply through the implementation of an active material such as Si offer a glimpse into the future of lighter and smaller batteries. Despite the advantages of the Si electrode, a number of challenges impede its commercialization. Many of these challenges are associated with the Si material’s severe volume expansion during lithiation. While the commercialized graphite electrode expands ~10–13% during lithium intercalation [13] , [14] , Si expansion amounts to nearly 300%, generating structural degradation and instability of the all-important solid-electrolyte interphase (SEI) [12] , [15] . Such instabilities ultimately shorten the battery life to inadequate levels. Degradation of the active material can be mitigated by incorporating materials <150 nm (ref. 16 ); however, research is yet to develop a practical solution to expansion-induced breaking of conduction channels, active material isolation and continuous SEI reformation [17] , [18] . Pioneering works have found some success in addressing material instability through the nanostructural design of electrode architectures capable of reducing expansion and its consequences [15] , [19] , [20] , [21] , [22] , [23] , [24] , [25] , [26] . The ultimate goal of such research is to incorporate a Si-based negative electrode into a lithium-ion full-cell, requiring the Si electrode to maintain a half-cell coulombic efficiency (CE) of >99.994% for 5,000 cycles [15] . These values, although somewhat unrealistic for current application needs, truly emphasize the importance of half-cell CEs to achieve a long-lasting LIB. Unfortunately, the electrode architectures presented in previous works [15] , [19] , [20] , [21] , [22] , [23] , [24] , [25] , [26] , despite providing significant improvements to Si electrode performance, lack the needed CEs largely because the volume change during Si alloying and de-alloying renders the SEI at the Si-electrolyte interface mechanically unstable. The SEI layer forms on the anode surface through reductive decomposition of the electrolyte during charging of the battery. Si anodes suffer extensively from a dynamic SEI that must reform each cycle as expansion during lithiation causes the layer to break [9] , [11] . Formation of the SEI consumes Li + and depletes electrolyte during every cycle [27] . In contrast to half-cells, which utilize a Li metal counter electrode with an effectively unlimited supply of Li + , full-cells have a limited supply of Li + provided by the cathode. It follows that the continuous breaking and reforming of the SEI layer quickly destroys the cell's cycling performance. Alternative electrolyte compositions [28] , [29] , [30] , [31] and active material surface treatments [32] have been studied in the effort to enhance SEI formation on high-capacity anode materials and improve half-cell CEs. In spite of these efforts, the CEs achieved throughout cycling are still insufficient for a long-lasting Si-based full-cell [31] , [33] , [34] , [35] or the methods employed to manufacture the full-cells introduce large excesses of Li + (>200%) into the system that serve to counterbalance the cell efficiency losses over long-term cycling [36] , [37] , [38] . In the effort to design next-generation electrolyte materials, room temperature ionic liquids (RTILs or ILs) are of particular interest due to their low volatilities, negligible vapour pressures, thermal stabilities, high-voltage stability windows and sufficient ionic conductivities [39] . Previous work has reported that RTILs, particularly those consisting of the pyrrolidinium (PYR 1 n + ) or 1-ethyl-3-methyl-imidazolium (EMIM + ) cation and the bis(trifluoromethanesulfonyl)imide (TFSI − ) or bis(fluorosulfonyl)imide (FSI − ) anion, are cathodically stable with popular negative electrode materials [36] , [40] , [41] , [42] including Si (refs 29 , 30 , 31 ). While the compatibility of ILs with such materials has been proven, a clear understanding of their electrochemical properties and interfacial chemistries has not yet been developed. Moreover, relatively little work has been dedicated to the study of the compatibility between RTIL electrolytes and Si-based nanocomposite electrodes, with all published work in this field, to date, investigating Si-RTIL systems in thin film type electrodes [29] , [30] , [31] . A combinatorial approach, one involving a mechanically resilient electrode architecture merged with an electrolyte capable of forming a favourable SEI, is the most promising option to integrate structural integrity with stable interfacial chemistry in a bulk type Si anode. To this end, we have designed a Si-RTIL system that exhibits a highly stable and resilient SEI, providing a solution to the drawbacks of the Si-anode and enabling the long-term operation of a lithium-ion full-cell with a bulk type Si-based anode. Through a systematic and comprehensive experimental matrix, we have studied the composition and structure of the SEI formed by an FSI − -based IL on our previously reported cyclized-polyacrylonitrile (cPAN)-based Si nanocomposite architecture (nSi-cPAN) [19] . Using experimental and theoretical data, we propose a mechanism for the formation of the SEI at the Si-RTIL interface and discuss the importance of CE in half-cell configurations. Most notably, this study is highlighted by the groundbreaking demonstration of the highly reversible cycling of a nSi-cPAN/Li(Ni 1/3 Mn 1/3 Co 1/3 )O 2 -(L333) full-cell using a PYR 13 FSI (1.2 M LiFSI) electrolyte. Half-cell electrochemical characterization The simple fabrication, scalability, low volume expansion and structural robustness of our previously reported nSi-cPAN architecture [19] make it an ideal candidate to merge with a suitable electrolyte system. In pursuit of a stable Si-electrolyte interface, the nSi-cPAN composite was cycled under galvanostatic conditions in RTILs comprising cation–anion combinations known for their cathodic stabilities against various negative electrode materials [29] , [30] , [31] , [36] , [40] , [41] , [42] . The cycling performances of the Si-based electrode in RTIL solutions, including PYR 13 FSI (1.2 M LiFSI), PYR 13 TFSI (0.6 M LiTFSI) and EMIMFSI (1.2 M LiFSI), were directly compared with the electrode performance in the commercial EC/DEC (1 M LiPF 6 ) electrolyte. The results of the preliminary cycling study are presented in Fig. 1 , demonstrating the exceptional cycling stability of the nSi-cPAN anodes in FSI − -based ILs and their unprecedented CE in the PYR 13 FSI system. The high CE manifested in the PYR 13 FSI (1.2 M LiFSI) electrolyte stabilizes after 8 cycles, with an average stable CE of 99.945% and a charge capacity retention of 76.7% after 100 cycles (blue profiles, Fig. 1a ). While exhibiting stable half-cell cycling, the lower average CE (98.451%) observed using an EMIMFSI (1.2 M LiFSI) electrolyte (orange profiles, Fig. 1b ) is ascribed to the instability of the EMIM + cation below 1.5 V (versus Li/Li + ) [41] . Such impressive data contrast that of the cycling behaviour of our nSi-cPAN electrode in a conventional organic electrolyte, which maintains only 45.2% of its initial charge capacity after 100 cycles with an average stable CE of 97.824% (red profiles, Fig. 1a ), and the rapid capacity fade and low-active material utilization in a TFSI − -based IL (green profiles, Fig. 1b ). The results obtained with organic electrolyte differ from our previous work [19] due to the absence of a voltage hold step during cycling, typically required to add stability and increase CE, and a higher-active material mass loading in this study (over double that of our previous work). The charge-discharge profiles generated by cycling the nSi-cPAN in each electrolyte solution are depicted in Supplementary Fig. 1 . 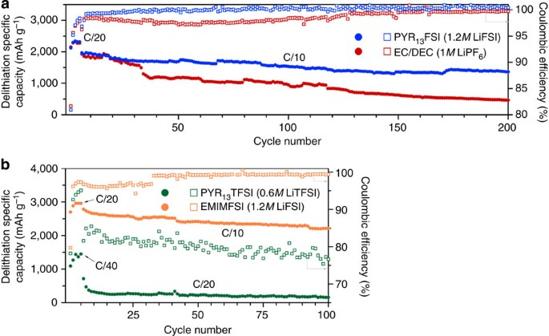Figure 1: Galvanostatic performance of various electrolyte systems with nSi-cPAN. (a) Specific capacities and coulombic efficiencies of nSi-cPAN electrode in PYR13FSI (1.2 M LiFSI) and EC/DEC (1 M LiPF6). (b) Specific capacities and coulombic efficiencies of nSi-cPAN electrode in PYR13TFSI (0.6 M LiTFSI) and EMIMFSI (1.2 M LiFSI) electrolyte systems. Cycling was carried out at room temperature in 2032 coin-type half-cells operated between 0.05 and 1 V (versus Li/Li+). Figure 1: Galvanostatic performance of various electrolyte systems with nSi-cPAN. ( a ) Specific capacities and coulombic efficiencies of nSi-cPAN electrode in PYR 13 FSI (1.2 M LiFSI) and EC/DEC (1 M LiPF 6 ). ( b ) Specific capacities and coulombic efficiencies of nSi-cPAN electrode in PYR 13 TFSI (0.6 M LiTFSI) and EMIMFSI (1.2 M LiFSI) electrolyte systems. Cycling was carried out at room temperature in 2032 coin-type half-cells operated between 0.05 and 1 V (versus Li/Li + ). Full size image The unparalleled CEs of the Si-PYR 13 FSI system are attributed to the formation of a highly stable SEI. We suggest that the breakdown of the ions present in the electrolyte solutions leads to varying SEI compositions dependent on the ionic make-up of the RTILs. We postulate that the interface formed by the decomposition products of the FSI − -based IL mitigates the continuous SEI formation experienced in organic electrolyte, and this proposal is substantiated by the longer cycling life of the Si-PYR 13 FSI half-cell ( Fig. 1a , blue profile), achieving an average CE of 99.97% in 200 cycles. Given the distinct incongruity of the nSi-cPAN electrode with the TFSI − -based electrolyte, the decomposition mechanisms and SEI compositions resulting from ILs comprising TFSI − and FSI − were explored using density functional theory (DFT) electronic structure methods. Theoretical simulation of RTIL reductive decomposition Mechanisms for the reductive decomposition of the FSI − and TFSI − anions on Li metal surfaces and in bulk solution have been examined in the literature [41] , [43] . Through parallel modelling treatments in different environments, we are able to compare potential SEI formation pathways in ILs containing both anions. The first type of theoretical study consists of cluster-based, localized basis calculations on isolated FSI − ( Fig. 2a ) and TFSI − ( Fig. 2c ) anions, and pairs of these ions ( Supplementary Fig. 2 ), mimicking one-electron reduction pathways in environments that do not react rapidly with the reduced species, including those inside the bulk liquid electrolyte or at cPAN interfaces. The second study consists of periodic boundary condition simulations of PYR 13 + /FSI − and PYR 13 + /TFSI − ion pairs on either a bare Li 13 Si 4 slab (010) surface, which mimics RTIL components that may have diffused into the more reactive electrode environments, or the same anions on model cPAN-coated Li 13 Si 4 surfaces. Similar initial bond-breaking pathways are obtained by these modelling treatments; thus, we will focus the following analysis on the study of ion pairs on a lithiated silicon surface. A detailed description of the localized basis calculations (first type of modelling study) is provided in the Supplementary Information and depicted in Supplementary Fig. 2 . To model our electrolyte molecules in direct contact with a pristine anode surface [43] , [44] , we first optimize PYR 13 + /FSI − and PYR 13 + /TFSI − ion pairs on the Li 13 Si 4 surface ( Fig. 2e,g , respectively). The same model surface was previously studied in the context of fluoroethylene carbonate (FEC) decomposition [45] and represents a low-potential anode surface with Si directly exposed to the liquid electrolyte, serving as an electron source that can readily reduce electrolyte molecules in its vicinity. 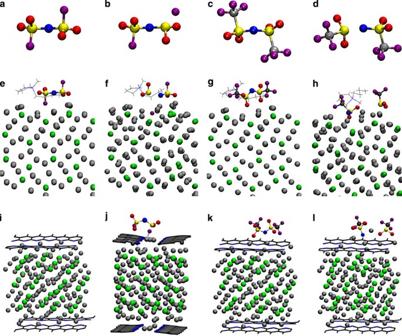Figure 2: Decomposition mechanism of FSI−and TFSI−anions on bare and cPAN-coated Li13Si4surface. Ball and stick models of the (a) FSI−anion (b) decomposed FSI2−radical di-anion, (c) TFSI−anion and (d) decomposed TFSI2−di-anion. DFT simulations of the (e) intact PYR13+/FSI−pair on bare Li13Si4, (f) decomposed PYR13+/FSI−pair on bare Li13Si4, (g) intact PYR13+/TFSI−pair on bare Li13Si4and (h) decomposed PYR13+/TFSI−pair on bare Li13Si4. In (e–h) excess electrons on FSI−or TFSI−are not added explicitly but come from Li13Si4. Ball and stick model of the (i) cPAN coating Li13Si4. DFT simulation of the (j) spontaneous decomposition of FSI−anion on cPAN-coated Li13Si4, (k) intact TFSI−anion on cPAN-coated Li13Si4and (l) decomposed TFSI−anion on cPAN-coated Li13Si4. Li, Si, C, O, N, S and F atoms are depicted as silver, green, grey, red, blue, yellow and purple spheres, respectively. The PYR13+cation is shown as a grey line diagram in the background of (e–h). All panels are optimized geometries except (f,h) which are AIMD snapshots atT=350 K. Figure 2: Decomposition mechanism of FSI − and TFSI − anions on bare and cPAN-coated Li 13 Si 4 surface. Ball and stick models of the ( a ) FSI − anion ( b ) decomposed FSI 2− radical di-anion, ( c ) TFSI − anion and ( d ) decomposed TFSI 2− di-anion. DFT simulations of the ( e ) intact PYR 13 + /FSI − pair on bare Li 13 Si 4 , ( f ) decomposed PYR 13 + /FSI − pair on bare Li 13 Si 4 , ( g ) intact PYR 13 + /TFSI − pair on bare Li 13 Si 4 and ( h ) decomposed PYR 13 + /TFSI − pair on bare Li 13 Si 4 . In ( e – h ) excess electrons on FSI − or TFSI − are not added explicitly but come from Li 13 Si 4 . Ball and stick model of the ( i ) cPAN coating Li 13 Si 4 . DFT simulation of the ( j ) spontaneous decomposition of FSI − anion on cPAN-coated Li 13 Si 4 , ( k ) intact TFSI − anion on cPAN-coated Li 13 Si 4 and ( l ) decomposed TFSI − anion on cPAN-coated Li 13 Si 4 . Li, Si, C, O, N, S and F atoms are depicted as silver, green, grey, red, blue, yellow and purple spheres, respectively. The PYR 13 + cation is shown as a grey line diagram in the background of ( e – h ). All panels are optimized geometries except ( f , h ) which are AIMD snapshots at T =350 K. Full size image After the geometric optimizations, which do not lead to chemical reaction, ab initio molecular dynamics (AIMD) simulations were initiated at 350 K. The FSI − anion rapidly decomposes within 1.2 ps ( Fig. 2f ). The S-F bond breaks first, releasing F − as shown in Fig. 2b , followed by detachment of the SO 2 group, which is expected to undergo further reaction with the anode surface and absorb a second electron. This rapid reaction cascade is reminiscent of the FSI − reactions predicted on Li metal surfaces. [43] TFSI − proves to be much less reactive than FSI − , staying intact on the Li 13 Si 4 surface for 21 ps at which point it decomposes ( Fig. 2d ). Neither of the two resulting fragments have a net magnetic moment, indicating that a two-electron reduction has occurred and formed SO 2 CF 3 − and NSO 2 CF 3 2− on the electrode surface ( Fig. 2h ). This prediction correlates with the initial majority product proposed by Markevich et al . [41] PYR 13 + remains inert throughout all of the aforementioned simulations. Further confirmation of these anion decomposition mechanisms is provided by also performing calculations on a cPAN-coated Li 13 Si 4 electrode model ( Fig. 2i ), which more accurately mimics the chemical environment of the experimental electrodes. Owing to the increment of the system size with cPAN coating, the PYR 13 + counter-ion was omitted in the decomposition simulations. Attempts to optimize FSI − on the surface lead to spontaneous breaking of the same S-F bond ( Fig. 2j ) as observed on the uncoated Li 13 Si 4 surfaces and in the cluster-based geometry. Figure 2j has been modified ( x -axis CCW rotation of about 90°) to display a better perspective of the FSI − anion on the cPAN surface. 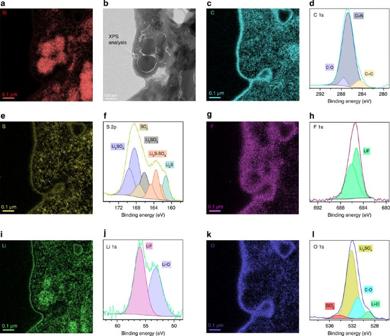Figure 3: Solid-electrolyte interphase composition of the Si-PYR13FSI system. (a) EELS elemental mapping of Si from (b) TEM micrograph of cycled nSi-cPAN electrode at the 16th delithiation along with EELS elemental mapping and XPS analysis of (c,d) carbon, (e,f) sulfur, (g,h) fluorine, (i,j) lithium and (k,l) oxygen, defining the elemental constitution and favored nucleation sites of the SEI formed. Supplementary Figure 3 provides the original (non-rotated) perspective of FSI − breakdown on the cPAN-coated Li 13 Si 4 surface. In contrast, TFSI − is readily optimized on the surface without bond-breaking reactions ( Fig. 2k ). Manually breaking the C-F bond and placement of the resulting F − in the Li-inserted cPAN gap lead to the reconstitution of the C-F bond, showing that the release of F − is not favourable. Instead, breaking S-N bonds leads to energetically favourable configurations ( Fig. 2l ). This is in accord with our calculations on bare Li 13 Si 4 surfaces and in the cluster-based geometry. To summarize our modelling study, we find that FSI − and TFSI − undergo quite different decomposition mechanisms on electrochemical reduction. FSI − rapidly releases F − , most likely forming LiF in the SEI, in combination with the release of SO 2 , suggesting the formation of an SEI composed of relatively small inorganic compounds. In contrast, TFSI − forms different products, including -SO 2 CF 3 groups, at much slower timescales. While some of the latter reduced fragments may eventually yield F − according to mechanisms proposed by Markevich et al . [41] , slower F − release, similar to the slow PF 6 − decomposition in organic electrolyte [44] , is expected by TFSI − . We speculate that the fast release of F − and SO 2 may be correlated to the high cycling performance exhibited by the Si-PYR 13 FSI system. This argument dovetails with earlier modelling studies of FEC decomposition, which show that FEC also rapidly releases F − to form LiF, as well as empirical data, showing favourable Si half-cell cycling behaviour when using FEC as an electrolyte additive in organic carbonate-based electrolyte [45] . It should be noted that FEC decomposition also releases large organic fragments [45] not found in the RTIL reduction pathway. Therefore, FEC and FSI − are not expected to yield identical SEI chemical compositions. To fully understand the unique role of the PYR 13 FSI as an electrolyte system and SEI former, we have investigated an EC/DEC/FEC (1.5 M LiPF 6 ) electrolyte system with our nSi-cPAN electrode architecture ( Supplementary Fig. 4 ). Despite the significant improvement in half-cell CEs (average stable CE of 99.216% in the first 100 cycles) compared with the EC/DEC (1 M LiPF 6 ) electrolyte, the CEs are still much lower than those exhibited by the PYR 13 FSI electrolyte system. These results illustrate the importance of the fast release of F − for the formation of LiF in combination with the formation of oxygen and sulfur-based compounds in the proposed SEI. PYR 13 FSI (1.2 M LiFSI) becomes, to the best of our knowledge, the first electrolyte system to enable such high half-cell CE values with a high-capacity anode material such as Si. Interfacial topography and composition By using electron energy loss spectroscopy (EELS) to study the elemental composition of the surface of nSi-cPAN particles during cycling (16th delithiation), we confirm our DFT predictions and gain insight into the elemental constitution and topography of the proposed SEI. Figure 3 displays high-resolution transmission electron microscopy (HRTEM) images of the cycled/delithiated nSi-cPAN cross-section ( Fig. 3b ) with EELS mapping of silicon ( Fig. 3a ), carbon ( Fig. 3c ), sulfur ( Fig. 3e ), fluorine ( Fig. 3g ), lithium ( Fig. 3i ) and oxygen ( Fig. 3k ). The well-defined silhouette of F coating the surface of the Si particles, in combination with the presence of Li, provides further evidence of an SEI composition containing LiF (refs 35 , 45 ), as proposed in literature [43] , [46] and found in our DFT simulations. Moreover, the clear mapping of O over the cPAN surface coating and evidence of S correlates with the proposed reaction of previously determined FSI − -breakdown products, such as SO 2 and LiO (refs 43 , 46 , 47 ). Similar analysis of a conventional Si-based electrode cycled in conventional, organic electrolyte shows no specific adherence of electrolyte decomposition products around the cycled Si particles ( Supplementary Fig. 5 ). Figure 3: Solid-electrolyte interphase composition of the Si-PYR 13 FSI system. ( a ) EELS elemental mapping of Si from ( b ) TEM micrograph of cycled nSi-cPAN electrode at the 16th delithiation along with EELS elemental mapping and XPS analysis of ( c , d ) carbon, ( e , f ) sulfur, ( g , h ) fluorine, ( i , j ) lithium and ( k , l ) oxygen, defining the elemental constitution and favored nucleation sites of the SEI formed. Full size image To elucidate the precise chemical composition of the proposed SEI, X-ray photoelectron spectroscopy (XPS) is utilized to verify the chemical bonding environments of the species observed physically with EELS and simulated through DFT. Alongside our EELS characterization, Fig. 3 displays the deconvolution of the C 1s ( Fig. 3d ), S 2p ( Fig. 3f ), F 1s ( Fig. 2h ), Li 1s ( Fig. 2j ) and O 1s ( Fig. 2l ) XPS spectra. Deconvolution of the C 1s spectrum shows a chemical environment consistent with that of the cyclized-PAN coating, dominated by the decomposition of and formation of ladder-like structures of thermally stable pyridine rings, C-N=C, and conjugation of the backbone, C=C (ref. 19 ). Deconvolution of the F 1s and Li 1s spectra provide direct chemical evidence of the formation of an SEI composition containing LiF and lithium-oxygen containing species (that is, LiO, LiOH), consistent with previous studies of SEIs formed by (fluorosulfonyl)imide-based RTILs [43] , [46] . Moreover, the deconvolution of the S 2p and O 1s spectra reveals evidence of the detachment and reaction of the SO 2 group from FSI − breakdown, confirming our DFT simulation and our EELS elemental mapping, in which the presence of sulfur- and oxygen-containing species was observed. The S 2p spectrum clearly shows the presence of SO 2 and its reaction on the surface of the particles to form sulfates, sulfites and sulfides, consistent with other works [43] , [46] , [47] . In addition to revealing the formation of sulfates, such as Li 2 SO 4 (ref. 47 ), and lithium-oxygen species, the deconvolution of the O 1 s spectra affirms the formation of carbon-oxygen components assigned to the reaction of O with the cPAN coating, suggesting the interaction of the SEI components with the coated electrode surface. Examination of the SEI formation mechanism via mass change To investigate the formation mechanism of the proposed SEI on the nSi-cPAN electrode, we turn to an examination of the mass changes on this interface during the first charge-discharge cycle using in situ electrochemical quartz crystal microbalance (EQCM). By monitoring mass increases and decreases on the electrode in real time during the first cycle, at which time the SEI forms its foundational structure, we gain an appreciation for the fragility of this interface in the conventional, organic electrolyte-based system while further proving the mechanical resilience of the Si-RTIL interface. 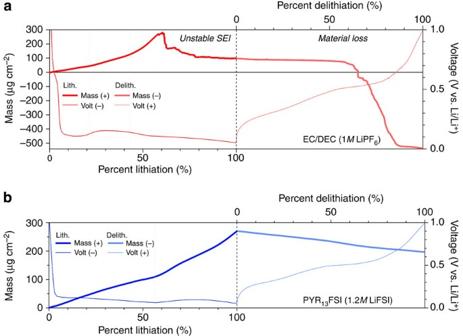Figure 4: Mass changes on the nSi-cPAN electrode during the first charge-discharge cycle. EQCM massograms obtained during the initial SEI formation cycle for the nSi-cPAN electrodes cycled in (a) conventional organic electrolyte and (b) PYR13FSI (1.2 M LiFSI) electrolyte, along with the voltage traces corresponding to each system. Figure 4 conveys EQCM massograms for the nSi-cPAN initial formation cycle in both organic electrolyte ( Fig. 4a ) and FSI − -based IL ( Fig. 4b ). Both systems reveal two very distinct behaviours during lithiation, as alluded to in our modelling study. The gradual rise in mass of about 43 μg cm −2 during the initial 20% of lithiation in both systems corresponds to the uptake of lithium by cPAN [21] , other non-faradaic processes and initial alloying of Li with Si. Figure 4: Mass changes on the nSi-cPAN electrode during the first charge-discharge cycle. EQCM massograms obtained during the initial SEI formation cycle for the nSi-cPAN electrodes cycled in ( a ) conventional organic electrolyte and ( b ) PYR 13 FSI (1.2 M LiFSI) electrolyte, along with the voltage traces corresponding to each system. Full size image Subsequently, the electrodes undergo rapid mass changes, attributed mainly to the decomposition of electrolyte and deposition of decomposition products on the electrode-electrolyte interface. The onset of these rapid mass changes are visible in the voltage trace of each system through the ‘potential overshoot’ phenomenon, a known artefact of electrolyte decomposition in EQCM experiments (further explained in the Supplementary Information ) [48] . The onset of this rapid mass change occurs earlier (20.5% lithiation) and at a significantly higher rate (reaching 73 g mol −1 of e − at 57.8% lithiation) in a conventional organic electrolyte. Mass change per mole of electrons (m.p.e., g mol −1 of e − ) values were extracted from data in Supplementary Fig. 6 and a more detailed analysis is provided in the Supplementary Information . This is owed to the lower electrochemical stability of the conventional organic electrolyte as compared with the PYR 13 FSI system, which has a voltage stability window of 7.31 V (ref. 49 ). The higher average m.p.e. in the conventional electrolyte system, along with the very slow F − release during EC/DEC (1 M LiPF 6 ) decomposition as proposed in literature [44] , suggests the formation of an SEI composed primarily of broken-down organic molecules. Conversely, the controlled mass gains, lower average m.p.e. (reaching 25 g mol −1 of e − after 56% lithiation and raising to 33 g mol −1 of e − towards the end of lithiation) and fast release of F − and SO 2 , as demonstrated earlier in this work, of the PYR 13 FSI (1.2 M LiFSI) electrolyte throughout lithiation substantiate our prediction of the formation of an SEI comprising relatively small inorganic compounds such as LiF and other sulfur- and oxygen-containing species. After reaching a critical mass of 282 μg cm −2 , the mass of the Si-conventional organic electrolyte system crashes. The crash in mass could be caused by a number of factors, including the severe volume expansion known to occur in this system causing breakage of the electrode matrix, and the build-up and rupturing of an unstable interfacial layer. During delithiation, contraction of the nSi-cPAN composite leads to further breakage of the electrode matrix and material loss. The inability of this system to exhibit stable mass changes corresponds to the incompatibility of Si with a conventional electrolyte. In contrast, the Si-RTIL system massogram exhibits more gradual mass growth and loss, with ~73% of the mass gained during initial lithiation remaining after delithiation. We attribute this behaviour to the irreversible formation of a stable interfacial layer on the Si electrode, manifesting stable cycling and high CEs throughout an impressive cycling life. Electrode morphology and volumetric expansion minimization While the theoretical and experimental data described provide insight into the formation mechanism and composition of the proposed SEI, we turn to a more comprehensive imaging examination to develop a direct understanding of the morphological effects of the PYR 13 FSI electrolyte on our Si-based electrode. Consistent with our previous work [19] , EELS and TEM reveal a thin, conformal coating of PAN on the nano-Si particles throughout the uncycled composite ( Fig. 5a,b ). Our previous work verified the mechanical advantages of the cPAN coating by analysing electrode cross-sections at different stages of cycle life, finding an overall electrode volumetric expansion of only 40% after full initial lithiation with an EC/DEC (1 M LiPF 6 ) electrolyte [19] . Through the same treatment of electrode cross-section samples taken before ( Fig. 5c ) and after ( Fig. 5d ) initial lithiation in a PYR 13 FSI (1.2 M LiFSI) electrolyte, we find the volumetric expansion of the nSi-cPAN composite to be just 17%. To further investigate this remarkable volume control, TEM micrographs were taken upon initial lithiation ( Fig. 5e,f ) and after the 16th delithiation ( Fig. 5g,h ). The TEM images of both the fully lithiated and cycled electrodes show no mechanical deficiencies or morphological changes within the Si particles or the composite structure. Most notably, after the 16th delithiation the Si-PYR 13 FSI system exhibits no severance of connection between the Si particles and cPAN network with striking preservation of the nano-Si spherical shape, contrasting the relatively poor nano-structural preservation of the same electrode in conventional electrolyte. [19] The impressive structural integrity of the Si-PYR 13 FSI system is undoubtedly linked to the system's cycling stability, suggesting that the Si-RTIL interface concurrently promotes favourable electrochemistry and structural resilience. 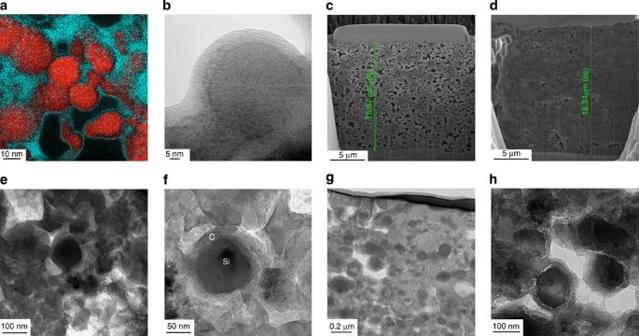Figure 5: Microstructure of nSi-cPAN and morphological effects of PYR13FSI IL on anode. (a) EELS elemental mapping of carbon (cyan) and silicon (red) and (b) TEM micrograph of the pristine nSi-cPAN electrode reveal a thin, conformal coating of PAN on the nano-Si particles throughout the uncycled composite. (c,d) FESEM images of electrode cross-sections before (c) and after (d) initial lithiation showing an electrode volume expansion of only 17%. (e–h) TEM micrographs of fully lithiated (e,f) and 16th delithiated (g,h) nSi-cPAN electrodes showing no mechanical deficiencies or significant morphological changes. Figure 5: Microstructure of nSi-cPAN and morphological effects of PYR 13 FSI IL on anode. ( a ) EELS elemental mapping of carbon (cyan) and silicon (red) and ( b ) TEM micrograph of the pristine nSi-cPAN electrode reveal a thin, conformal coating of PAN on the nano-Si particles throughout the uncycled composite. ( c , d ) FESEM images of electrode cross-sections before ( c ) and after ( d ) initial lithiation showing an electrode volume expansion of only 17%. ( e – h ) TEM micrographs of fully lithiated ( e , f ) and 16th delithiated ( g , h ) nSi-cPAN electrodes showing no mechanical deficiencies or significant morphological changes. Full size image As previously mentioned, the ultimate goal of much electrochemical materials research is to incorporate high-capacity electrodes into a lithium-ion full-cell. Up to this point in our study, we have provided in-depth characterization of the Si-PYR 13 FSI system and proposed a mechanism for the system’s stability through a remarkably robust SEI. The most dependable means of substantiating our claim of a stable SEI is to demonstrate the long-term cycling of a full-cell incorporating the Si-PYR 13 FSI system. Combining this work and our previous study of the compatibility between PYR 13 FSI electrolytes and the L333 cathode chemistry [49] , we have built nSi-cPAN/PYR 13 FSI (1.2 M LiFSI)/L333 LIBs capable of maintaining high energy-densities for an exceptionally long cycling life (see Methods for details on full-cell fabrication). 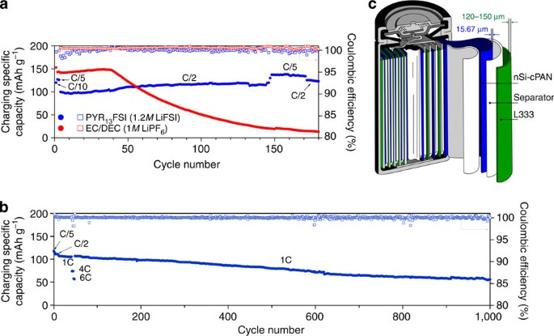Figure 6: Full-cell electrochemical performance of nSi-cPAN/L333 with PYR13FSI versus EC/DEC electrolyte systems. (a) Specific charge capacities and coulombic efficiencies of nSi-PAN/L333 full-cells assembled with PYR13FSI (1.2 M LiFSI) and conventional EC/DEC (1 M LiPF6) electrolytes. (b) nSi-cPAN/PYR13FSI/L333 full-cell rate study and long-term cycling. (c) Mock-up of a commercial 18650 cell showing the possibility of incorporating more electroactive material due to the relatively thin nSi-cPAN electrode. Cycling was carried out at room temperature in 2032 coin-type half-cells operated between 2.0 and 4.15 V (versus Li/Li+). Figure 6a compares the performance of nSi-cPAN/L333 full-cells assembled with conventional EC/DEC (1 M LiPF 6 ) and PYR 13 FSI (1.2 M LiFSI) electrolytes. Both cells presented in Fig. 6a contain the same electrode mass loading on both cathode and anode (within 10%) and were operated and controlled under the same parameters for fair comparison. All of the full-cells presented in this work were preconditioned to accurately control the amounts of Li in the cell and state of charge of the electrodes (see Methods for details on full-cell fabrication), allowing for accurate comparison between cells. Initial charge capacities of 143.21 and 127.10 mAh g −1 (all full-cell specific capacities are normalized with respect to total active material mass) were observed at the C/5 rate for the EC/DEC (1 M LiPF 6 ) and PYR 13 FSI (1.2 M LiFSI) LIBs, respectively. The difference in initial capacity is attributed to the higher resistance of the RTIL electrolyte, though this limitation is countered by unparalleled cycling stability. After 35 cycles, the cell cycled in carbon-based electrolyte degrades rapidly. The degradation, ascribed to low half-cell CEs with an average irreversible charge loss of 2.31% per cycle ( Fig. 1a , red profile), occurs as the system exhausts its supply of Li through continuous SEI breaking and reformation. In contrast, the cell cycled in PYR 13 FSI (1.2 M LiFSI) electrolyte shows remarkable stability, attributed to the high half-cell CEs, with an average irreversible charge loss of just 0.076% for the first 100 cycles ( Fig. 1a , blue profile) followed by negligible Li consumption, providing an average full-cell charge capacity of 110.98 mAh g −1 at a rate of C/2 ( Fig. 6a , blue profile). To further investigate the SEI stability of the Si-PYR 13 FSI system, a full-cell was cycled for longevity with a brief rate study. Figure 6b depicts the nSi-cPAN/PYR 13 FSI (1.2 M LiFSI)/L333 cell run for 1,000 cycles delivering 107.33, 74.70 and 58.26 mAh g −1 at rates of 1C, 4C and 6C, respectively (1C rate capacity value pertains to the average of the first 40 cycles at this rate). Figure 6: Full-cell electrochemical performance of nSi-cPAN/L333 with PYR 13 FSI versus EC/DEC electrolyte systems. ( a ) Specific charge capacities and coulombic efficiencies of nSi-PAN/L333 full-cells assembled with PYR 13 FSI (1.2 M LiFSI) and conventional EC/DEC (1 M LiPF 6 ) electrolytes. ( b ) nSi-cPAN/PYR 13 FSI/L333 full-cell rate study and long-term cycling. ( c ) Mock-up of a commercial 18650 cell showing the possibility of incorporating more electroactive material due to the relatively thin nSi-cPAN electrode. Cycling was carried out at room temperature in 2032 coin-type half-cells operated between 2.0 and 4.15 V (versus Li/Li + ). Full size image It is noted that the PYR 13 FSI RTIL strengthens the performance of a range of previously developed Si-based anode architectures, not just those containing PAN ( Supplementary Fig. 7 ). Moreover, preliminary study of the high-temperature performance of the Si-RTIL system has also yielded promising results ( Supplementary Fig. 8 ), suggesting that the SEI formed by PYR 13 FSI is stable even at elevated temperature. It is understood that the overall energy density of LIBs is limited by the capacity of the positive electrode. While this study demonstrates a significant advancement in the study of LIB anode materials, a high-capacity cathode compatible with the Si-PYR 13 FSI pair should be developed to truly realize the benefits of the system. In spite of limitations introduced by the battery cathode capacity, we propose that introducing the Si-PYR 13 FSI system into a commercial 18650 cell configuration, as shown in Fig. 6c , would allow for incorporation of more electroactive material due to the relatively thin nSi-cPAN electrode. On the basis of a commercial battery with a 2 mAh cm −2 areal capacity and nominal voltage of 3.6 V, utilizing the nSi-cPAN electrode, which is <1/4 the thickness of a conventional graphite electrode and needs <1/5 electroactive material to achieve similar battery capacities, would allow for at least a 35% increase in overall battery capacity and thus the production of a higher energy-density LIB. Validated by impressive cycling data and a combination of theoretical and experimental results, our approach to developing a stable high energy-density anode-electrolyte system represents important progress towards a safer, higher-performance secondary LIB. Electrode and electrolyte preparation nSi-cPAN and Li(Ni 1/3 Mn 1/3 Co 1/3 )O 2 electrodes were fabricated according to our procedures described in refs 19 and 49 , respectively. Active material mass loading on both cathode and anode is at least double that of the referenced works. Ionic liquid electrolytes were provided by Boulder Ionics Corporation (USA) and scanned for halide impurities. Impurities (F − , Cl − , Br − , SO 4 − ) were quantified using a Dionex ICS-1100 chromatograph, calibrated for sensitivities as low as 1 p.p.m. Ion chromatography was performed on all ionic liquids and lithium salts used in this work, and the total impurity content of every solution was calculated based on the mass percentage of electrolyte component in the total mass of electrolyte. The solutions contained <20 p.p.m. (w/w) of moisture and <10 p.p.m. (w/w) of halide and metal-ion impurities. One molar LiPF 6 in ethylene carbonate:diethyl carbonate (50:50, Soulbrain) was used as a conventional organic electrolyte. Electrochemical characterization Electrochemical measurements were carried out using an Arbin BT2000 battery test station. All half-cells were assembled using our prepared nSi-cPAN electrodes as the working electrode and lithium metal foil as the counter electrode. The separator was a glass micro-fibre disc (Whatman GF/F) and the shell was a stainless steel CR2032 coin cell (Pred Materials). The electrolyte systems utilized were EC/DEC (1 M LiPF 6 ), PYR 13 FSI (1.2 M LiFSI), PYR 13 TFSI (0.6 M LiTFSI) and EMIMFSI (1.2 M LiFSI). We used a constant current (CC) testing scheme to cycle our half-cells. No voltage holds were utilized during cycling (lithiation or delithiation), preventing the currents applied to relax and supply/remove extra Li + , to highlight the true values of the cells’ coulombic efficiencies for each respective current. The half-cells were discharged (lithiated) and charged (delithiated) with various cycling currents (where a C/10 rate is equivalent to 353.6 μA cm −2 ) between 0.05 and 1 V (versus Li/Li + ). Electrochemical measurements of half-cells were all normalized based on the mass of Si-active material in each electrode (typically 1.1–1.3 mg). We used a constant current constant voltage (CCCV) testing scheme to cycle our full-cells. The full-cells were discharged and charged with various cycling currents (where a C/2 rate is equivalent to 502.9 μA cm −2 for the full-cells in Fig. 6a and 197.3 μA cm −2 for the full-cell in Fig. 6b ) between 2 and 4.15 V (versus Li/Li + ). Electrochemical measurements of full-cells were all normalized with respect to total mass of electro-active material in both cathode and anode electrodes (typically 7–9 mg). Electronic structure calculations Two types of calculations were conducted as mentioned in the main text. A detailed description of both the static cluster-based calculation and ab initio molecular dynamics (AIMD) simulations with a bare or cPAN-coated Li 13 S 4 slab, and further discussions of the theoretical literature, can be found in the Supplementary Information . cPAN is modelled as graphene strips terminated with C–N=C bonds [19] , with a gap between the terminal sp 2 -hybridized N atoms to allow for the intercalation of lithium, necessary for the Li + transport ( Fig. 2i ). Morphological characterization FIB (FEI, NOVA200 dual beam system) equipped with a mobile air-lock chamber was used for TEM sample preparation [50] . TEM and EELS analysis were performed with a FEI Tecnai F20 operated at 200 keV. A detailed description of our TEM and EELS characterization procedures can be found in ref. 51 . X-ray photoelectron spectroscopy XPS spectra were obtained on an AXIS His 165 and ULTRA spectrometer (Kratos) to determine the bonding configurations and chemical state of the elements present on the surface of the cycled nSi-cPAN particles. Argon milling was utilized for depth profiling (20 nm of depth). Electrochemical quartz crystal microbalance Similar to the electrode preparation for the coin-cell testing, nSi-cPAN films were coated on 1 inch diameter Pt 5-MHz resonating quartz crystals (Stanford Research Systems; SRS). The electrochemically active area in the cell was determined to be 1.359 cm 2 , based on the Pt pattern on the crystal. To mitigate error associated with frequency measurements using thick films on quartz crystals, all nSi-cPAN films were prepared with thicknesses under 10 μm. The crystals were placed in a SRS QCM200 crystal holder. The holder was modified with PEEK insulation so that a standalone cell, with a volume of 2.5 ml, could be enclosed with a lid. The ceiling of the cell was lined with a Li foil counter electrode and connected to a copper wire. All current and potential parameters were consistent with the electrochemical characterizations of the coin-cells. Full-cell fabrication Full-cells were fabricated from pre-conditioned electrodes selected based on deliverable capacity. Calculated from the active material mass, nSi-cPAN anodes were fabricated and matched with L333 cathodes such that the total anode capacity was ~160% of that of the cathode capacity. Both electrodes were then pre-conditioned: the anodes were allowed to run for 10 charge-discharge cycles in a half-cell configuration and were stopped after full lithiation, while the cathodes were allowed to run for 3 charge-discharge cycles in a half-cell configuration and were stopped after full delithiation. The half-cells were then disassembled and the electrodes were used to fabricate 2032 coin-cell (Al-clad cathode cup) type full-cells. This method of pre-conditioning allows for full control of the amount of lithium in the system. How to cite this article: Molina Piper, D. et al . Stable silicon-ionic liquid interface for next generation lithium-ion batteries. Nat. Commun. 6:6230 doi: 10.1038/ncomms7230 (2015). Dislaimer Any opinions, findings and conclusions or recommendations expressed in this material are those of the author(s) and do not necessarily reflect the views of the National Science Foundation.